A balanced measure shows superior performance of pseudobulk methods in single-cell RNA-sequencing analysis 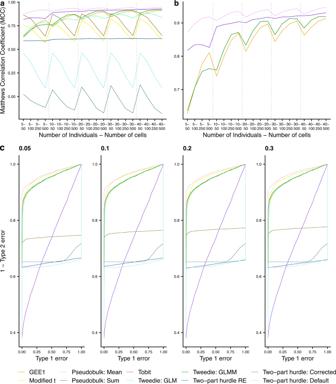Fig. 1: Performance of the analysed models. a,bgive the average Matthews correlation coefficient from the 20,000 iterations; 50 runs for each of the 5–40 individuals and 50–500 cells at ap-value cut-off of 0.05 on 10,000 genes.ashows all benchmarked models whereasbfocuses on the top four approaches.cgives the receiver operating characteristics (ROC) curve across 50 runs each for different proportions of simulated differentially expressed genes (DEGs)—0.05, 0.1, 0.2, 0.3. Twenty individuals were simulated for case and controls, each with 100 cells. The performance split by each iteration is given in Supplementary Table2. The different models are pseudoreplication approaches; ‘Modified t’, ‘Tobit’, ‘Two-part hurdle: Default’, ‘Two-part hurdle: Corrected’, ‘GEE1’, ‘Tweedie: GLM’, pseudobulk approaches; ‘Pseudobulk: Mean’, ‘Pseudobulk: Sum’ and mixed model approaches; ‘Tweedie: GLMM’ and ‘Two-part hurdle: RE’. More detail on these models is given in Supplementary Table1. Source data are provided as a Source Data file. Further information on research design is available in the Nature Portfolio Reporting Summary linked to this article.